Transcriptome meta-analysis of lung cancer reveals recurrent aberrations inNRG1and Hippo pathway genes Lung cancer is emerging as a paradigm for disease molecular subtyping, facilitating targeted therapy based on driving somatic alterations. Here we perform transcriptome analysis of 153 samples representing lung adenocarcinomas, squamous cell carcinomas, large cell lung cancer, adenoid cystic carcinomas and cell lines. By integrating our data with The Cancer Genome Atlas and published sources, we analyse 753 lung cancer samples for gene fusions and other transcriptomic alterations. We show that higher numbers of gene fusions is an independent prognostic factor for poor survival in lung cancer. Our analysis confirms the recently reported CD74-NRG1 fusion and suggests that NRG1 , NF1 and Hippo pathway fusions may play important roles in tumours without known driver mutations. In addition, we observe exon-skipping events in c-MET, which are attributable to splice site mutations. These classes of genetic aberrations may play a significant role in the genesis of lung cancers lacking known driver mutations. Lung cancer is the leading cause of cancer-related deaths [1] , [2] and is histologically classified as either non-small cell lung cancer (NSCLC) or small cell lung cancer (SCLC). NSCLC accounts for 80% of all lung cancers with lung adenocarcinoma (LUAD) and squamous cell carcinoma (LUSC) representing the major subtypes and large cell lung cancer (LCLC) and lung adenoid cystic carcinomas (LACC) representing the minor subtypes. LUAD are increasing in incidence worldwide [3] . Lung cancers poor overall 5-year survival rate (~15%) is primarily attributable to late diagnosis when curative surgery is no longer an option [2] . Genomic analyses of LUAD have revealed mutations in many known oncogenes and tumour suppressor genes including KRAS , EGFR , TP53 , CDKN2A and STK11 (ref. 4 ). These tumours also harbour low-frequency copy number alterations including ERBB2 amplification, which is targetable with herceptin [5] . Alterations in oncogenes such as KRAS , EGFR , ALK and MET influence tumour formation and maintenance, and are considered ‘drivers’ in a subset of NSCLCs, yet in a substantial patient population the driver aberrations are yet to be identified (that is, ‘driver mutation unknown’) [6] . Recent analyses by The Cancer Genome Atlas (TCGA) of both LUSC [7] and LUAD [8] revealed recurrent mutations and copy number alterations in genes that are present in both subtypes and are also specific to each. The histologic and molecular heterogeneity observed in lung cancer underscores the difficulties in developing effective therapies for patients. Patients with EGFR mutations show responsiveness to epidermal growth factor receptor (EGFR) inhibitors, which are often not durable [9] . In addition to driver somatic gene mutations, oncogenic gene fusions including the EML4-ALK fusion gene have been identified in ~4% of LUAD [10] . This fusion protein links the amino-terminal portion of echinoderm microtubule-associated protein-like 4 (EML4) with the intracellular signalling portion of a receptor tyrosine kinase, the anaplastic lymphoma kinase (ALK). The EML4-ALK translocation is mutually exclusive with EGFR and KRAS mutations, an indicator of therapeutic responsiveness to ALK inhibitors, [10] and tumours with this translocation also have fewer TP53 gene mutations [11] . Additional gene fusion events have now been identified in LUAD, including KIF5B-ALK [12] , ROS1 (ref. 13 ) and RET (refs 14 , 15 ) gene fusions. KIF5B-ALK fusion-positive lung cancers may respond to ALK inhibitors, whereas RET fusions may be treated using drugs that target this kinase [16] . We previously identified NFE2 and FGFR3 gene fusions in a subset of lung cancers [17] , [18] . In this study, we perform transcriptome meta-analysis on a data compendium assembled by combining 153 primary NSCLCs that we sequenced, with 521 NSCLCs from the TCGA and 79 samples from a published report [19] . The highly heterogeneous lung cancer gene fusion landscape is dominated by low recurrence and private fusions. We demonstrate that the number of fusions in a sample is an independent prognostic factor for poor survival. We found gene fusions affecting core members of the Hippo pathway, Neurofibromatosis 1 ( NF1 ) and Neuregulin 1 ( NRG1 ) genes, along with the recently reported CD74-NRG1 fusion variant [20] , [21] , [22] and c-MET exon-skipping event [23] . On integrating fusion, mutation and outlier expression data, these events collectively account for ~16% of driver-negative lung cancer samples. Analysis work flow and mutation landscape of NSCLC subtypes We sequenced messenger RNA from 153 samples representing major (LUAD and LUSC) and minor (LULC and LACC) subtypes of NSCLC using strand-specific, RNA paired-end sequencing (RNASeq). Our ‘UMICH cohort’, samples included 67 LUAD, 36 LUSC (64 stage I, 17 stage II and 22 stage III patients), 9 LCLC, 11 LACC, 24 lung cancer cell lines and 6 matched non-malignant lung samples. 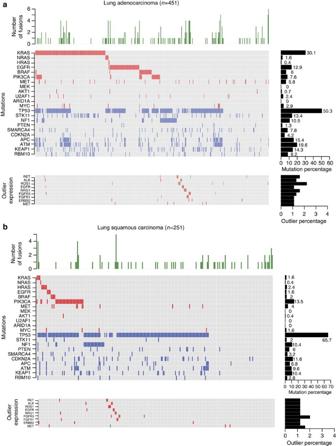Figure 1: The gene fusion and mutational landscape of lung cancers. (a) LUAD (n=451). (b) LUSC (n=251). Top panels represent histograms depicting the number of high-quality gene fusions identified in each sample. Central panels denote the presence or absence of activating mutations in known oncogenes (red), deleterious mutations in tumour suppressors (blue) and no aberration (grey). Samples are represented in columns and genes in rows. Right middle panel are bar plot summarizing the number of samples harbouring activating or deleterious mutations for each gene. Bottom panels indicate samples harbouring both known and novel gene fusions (in green) involving either receptor kinase genes orNRG1. Samples in red indicate outlier expression pattern observed in the respective genes. Cohorts of additional NSCLCs including LACC (n=11) and large cell carcinomas (n=9) were also analysed and are included inSupplementary Table 2. Eighty-two patients were heavy smokers (>20 pack-years), 13 were light smokers (defined by <20 pack-years) and smoking status of 15 patients was unknown ( Supplementary Table 1 ). The median smoking pack-years was 45 (range, 2–300). The average follow-up was 5.05 years. Sample acquisition details are provided in the Methods section. To increase the power of our analysis and to discover recurrent fusions, we included two publically available NSCLC data sets from TCGA and Korean LUAD (SEOUL cohort) studies [19] , and assembled an RNASeq cohort that totaled 753 patient tumours. The TCGA cohort included 305 LUAD and 216 LUSC samples (250 stage I, 112 stage II, 101 stage III and 19 stage IV cases, and 39 with unknown stage). The combined cohort included 451 LUAD, 251 LUSC, 9 LCLC, 11 LACC and 24 NSCLC cell lines, making this the most comprehensive RNA-sequencing cohort of lung cancers assembled to date. A description of the cohort assembly and sample clinical–pathological information is presented in the Methods section and summarized in Supplementary Table 1 . The available clinical information including smoking history is presented in Supplementary Data 1 . We developed the analysis pipeline, depicted in Supplementary Fig. 1 , thus assessing gene fusions among all 753 patients in the combined cohort and for integration with mutation and clinical information (see Methods for details). For each sample, we determined the mutation status of oncogenes and tumour suppressors known to play a role in lung cancer [6] and reflected the previously reported mutational landscape of LUAD and LUSC ( Fig. 1 ) [4] , [5] , [7] . KRAS was mutated in 30.1% and 1.6% of LUAD and LUSC, respectively; EGFR in 13% and 1.6% of LUAD and LUSC, respectively; BRAF in 8% and 3.2% of LUAD and LUSC, respectively; and PIK3CA in 7.6% and 13.5% of LUAD and LUSC, respectively. As previously reported [4] , [5] , [7] , TP53 mutations are common in both LUAD and LUSC patients, 50.3% and 65.7%, respectively ( Fig. 1 ). The mutations identified among select genes in the characterized cell lines are summarized in Supplementary Fig. 2 . Figure 1: The gene fusion and mutational landscape of lung cancers. ( a ) LUAD ( n =451). ( b ) LUSC ( n =251). Top panels represent histograms depicting the number of high-quality gene fusions identified in each sample. Central panels denote the presence or absence of activating mutations in known oncogenes (red), deleterious mutations in tumour suppressors (blue) and no aberration (grey). Samples are represented in columns and genes in rows. Right middle panel are bar plot summarizing the number of samples harbouring activating or deleterious mutations for each gene. Bottom panels indicate samples harbouring both known and novel gene fusions (in green) involving either receptor kinase genes or NRG1 . Samples in red indicate outlier expression pattern observed in the respective genes. 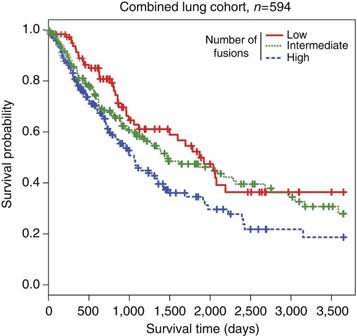Figure 2: Gene fusion numbers correlates with lung cancer prognosis. Kaplan–Meier analysis for the combined cohort of lung cancer samples (n=594) with low (0–7) (n=124), intermediate (8–16) (n=237), or high (≥17) (n=233) number of fusions (likelihood ratio testP=0.008). Samples with high number of fusions have worse prognosis (Cox survival analysisP=0.005). Individual Kaplan–Meier analyses with LUAD and LUSC samples are found inSupplementary Fig. 4a,b, respectively. Cohorts of additional NSCLCs including LACC ( n =11) and large cell carcinomas ( n =9) were also analysed and are included in Supplementary Table 2 . Full size image In addition to the major NSCLC subtypes, we profiled 9 LCLC and 11 LACC, also called lung colloid carcinoma, a rare subtype. In LCLC, we found one sample with KRAS activating mutation, three with TP53 missense mutations and four without mutations in known lung cancer genes ( Supplementary Table 2 ). The pattern observed in LCLC is consistent with a recent report [24] supporting their reclassification into either LUAD or LUSC based on shared genetic aberrations. In LACC, despite the small sample size, we observed a higher frequency of RAS/RAF pathway mutations (72%, 8/11) compared with the major NSCLC subtypes ( Supplementary Table 2 ). The mutations were mutually exclusive, where five samples with KRAS mutations had KRAS G12C, G12V, G13C, G12D, Q61H variants, respectively, while BRAF V600E , HRAS Q61L and NRAS Q61R were observed in three independent samples. Interestingly, the samples with NRAS Q61R and KRAS G13C also had mutations in TP53 R141C, R141L and KIT M537L . MET T1010I variation was also observed in the NRAS -mutated sample. Although two LACC samples had no mutations reported in COSMIC, one sample harboured an IDH1 V178I variant. Interestingly, MYB-NF1B gene fusions were absent in the LACC, unlike the salivary gland ACC where it occurs in 57% of cases [25] . Likewise, KRAS mutations were common in LACC, but none were detected in the 60 salivary gland ACCs sequenced recently [25] . However, in the salivary gland ACC cohort, a potential driver HRAS non-synonymous mutation was noted to be mutually exclusive with MYB gene fusion. Another recent study identified activating BRAF and HRAS mutations in breast adenoid cystic carcinoma samples that were a distinct subset of triple-negative breast cancers [26] , [27] . Hence, the previous report on breast adenoid cystic carcinoma and our results here on LACC have identified distinct ACC subsets that harbour activating RAS/RAF mutations but lack MYB fusions that are primarily found in head and neck ACC, revealing differences in underlying molecular events despite histological similarities. Owing to the small cohort size and lack of significant fusion events in LCLC and LACC samples, these cohorts were excluded from the fusion analysis presented below. NSCLC fusion landscape To generate comparable results across samples from different cohorts, we developed a consistent data-driven gene fusion prediction pipeline and analysis workflow shown in Supplementary Fig. 1 (also see Methods). We detected 6,348 unique fusions among the 733 samples for an average of 13 fusions per tumour sample (range: 0–67). Although both LUAD and LUSC had a comparably high single-nucleotide mutation rate of 8.1 mutations per Mb [5] , [7] , they differed in the average number of fusions per sample with 11 fusions in LUAD and 17 in LUSC (Student’s t -test P <2.2e−16). 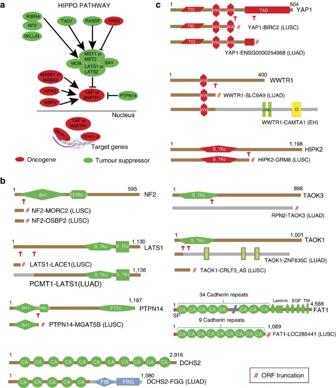Figure 3: Gene fusions among the Hippo pathway genes in lung cancer. (a) Schematic representation of core and associate members of the Hippo pathway adapted from Harveyet al.29Potential tumour suppressors are represented in green, whereas potential oncogenes are indicated in red. Phosphorylation of YAP or TAZ by LATS retains them in the cytoplasm and hinders their transcriptional regulation. (b) Fusions in putative oncogenes of the Hippo pathway. (c) Fusions in putative tumour suppressors of the Hippo pathway. For all fusion schematics represented, the wild-type Hippo pathway protein domain structure is presented first, numbers indicate total amino acids and domain names are abbreviated. Red arrows show the fusion junctions and red # symbol indicate protein truncation due to out-of-frame ORFs from fusion transcript analysis. The schematic of the previously reported TAZ-CAMTA1fusion in epithelioid hemangioendothelioma (EH)42is also displayed. Protein abbreviations: MST1/2, STE20-like protein kinase; LATS1/2, large tumour suppressor homologue kinase; YAP1, Yes-associated protein 1; WWTR1, ww-domain containing transcription regulator 1; TEAD, TEA-domain family; HIPK2, homeodomain interacting protein kinase 2; TAOK1/3, TAO kinase; FAT1, FAT atypical cadherin 1; DCHS2, dachsous cadherin-related 2; PTPN14, protein tyrosine phosphatase, non-receptor type 14. Domain abbreviations: B4, Band 4.1 homologues; FERM_C, FERM C-terminal PH-like domain; S_TKc, serine/threonine protein kinases, catalytic domain; PTPc, protein tyrosine phosphatase, catalytic domain; CA, cadherin repeats; FIB, fibrinogen; FBG, fibrinogen-related domains; WW, domain with 2 conserved Trp (W) residues; TID, TEAD interacting domain; TAD, transactivation domain; ANK,ankyrin repeats; IQ, short calmodulin-binding motif; EGF, epidermal growth factor-like domain; ZnFC2H2, zinc finger; TM, transmembrane domain. We did not observe a statistically significant difference in average number of fusions among heavy and light smokers (LUAD Student’s t -test P =0.06; LUSC Student’s t -test P =0.59) among different clinical stages and regardless of the tumour type ( Supplementary Table 3 ). Tumours with missense or nonsense mutations in TP53 showed greater average number of fusions compared with samples with wild-type TP53 ( Supplementary Fig. 3a,b , P =0.001). As most LUSC have somatic mutations in TP53 (ref. 7 ), this difference is consistent with the average number of fusions between LUAD and LUSC samples. In LUAD, we observed a significant correlation between the presence of oncogenic mutations (for example, KRAS -activating mutations), TP53 deleterious mutations (stop codon or splice site mutations) and the number of fusions (Fisher’s exact test P =0.008). We could not determine whether a similar correlation exists in LUSC due to the low incidence of mutations in KRAS , EGFR or other oncogenes in the samples. Number of fusions is associated with prognosis We investigated the relationship between the number of fusions present in a tumour and patient prognosis. Patients in our combined cohort were first classified into three fusion categories based on distribution percentiles as low (0–7), intermediate (8–17) or high (≥18), and then a 10-year Kaplan–Meier survival analysis was performed. Patients with high number of fusions had significantly shorter median overall survival (35.6, 95% confidence interval (CI) 27.2–43.9) compared with patients with intermediate (49.5, 95% CI 23.9–75.1) or low number of fusions (62.3, 95% CI 44.6–80.1; likelihood ratio test P =0.008 Fig. 2 ). We observed similar results both for LUAD and LUSC when analysed independently ( Supplementary Fig. 4a,b ). 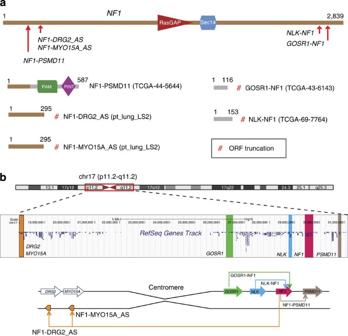Figure 4: Inactivating gene fusions ofNF1in lung cancer. (a) NF1 protein schematic and the observed fusion breaks (red arrows) in the index cases are displayed on top. RecurrentNF1fusions with partners (GOSR1,PSMD11,NLK,DRG2antisense andMYO15Aantisense) resulted in loss of theNF1gene as illustrated by the corresponding fusion protein structure below. Index samples are indicated in parenthesis and the numbers over the protein schematic indicate total amino acids. Red # symbol indicate protein truncation due to out-of-frame ORFs from fusion transcript analysis. (b) UCSC browser view of genomic location ofNF1gene and its fusion partners (top). Schematic representation of various NF1 rearrangements on chromosome 17 identified in lung cancer (bottom). Statistically significant clinical covariates in the univariate Cox model ( Supplementary Table 4 ) were used in the multivariate analysis to examine the prognostic value of fusion number. 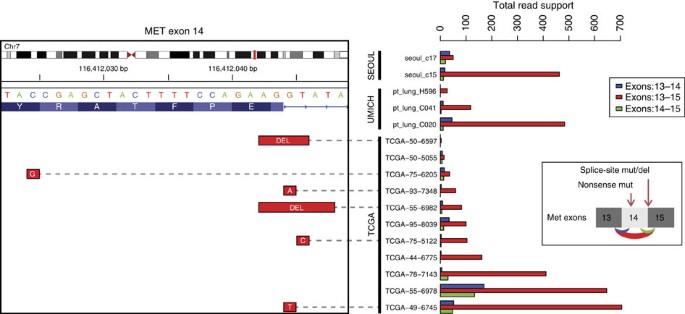Figure 5: Recurrent activatingMETexon-skipping events. Right panel: an activatingMETexon-14 skipping event was observed in a total of 15 tissue samples across all three cohorts. The total reads supporting each splice variant exon13–14 (blue), exon13–15(red) and exon14–15 (green) are represented in the bar plot on the right. In 5 out of 11 TCGA samples where DNA mutation data were available, skipping ofMETexon-14 was accompanied by a mutation affecting the splice donor site adjacent to position D1010 (illustrated inset on the right). In addition, one sample harboured a non-sense mutation g.chr7:116412024C>Gp.Y1003*, which accompanied exon-14 skipping. Left panel: IGV browser view of splice site deletions/mutations in the corresponding samples. Strikingly, a high fusion incidence was independently associated with worse overall survival (hazard ratio=1.56, 95% CI 1.13–2.15, P =0.007, Supplementary Table 5 ) after adjusting for gender and disease stage. 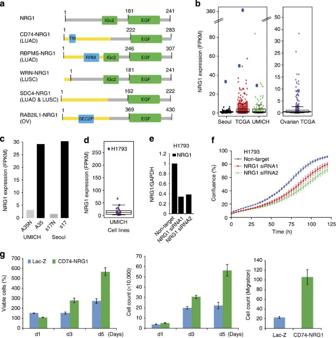Figure 6: RecurrentNRG1rearrangements in lung cancer. (a) Recurrent fusions involving NRG1 as a 3′-partner were detected in lung adenocarcinoma and lung squamous carcinoma in the three cohorts included in this study. Schematic representation of functional domains present in the NRG1 fusion proteins namelyCD74-NRG1;RBPMS-NRG1(LUAD),WRN-NRG1(LUSC),SDC4-NRG1(LUSC) andRAB2IL1-NRG1(ovarian cancer from TCGA) compared with the wild-typeNRG1(top). The receptor-binding EGF domain is preserved in all fusions. TM, transmembrane domain; RRM domain; IGc2 domain; SEC2P domain. (b) Analysis of RNASeq expression values revealed outlierNRG1mRNA expression in all index cases (large blue dots) within each cohort. (c) HighNRG1mRNA expression driven by the fusion event in the index tumour tissue compared with matched normal, in both an LUAD patient in the University of Michigan and Seoul cohorts. (d) Box plot showing outlier expression ofNRG1in H1793 in the University of Michigan lung cell line cohort. (e) Two independent small interfering RNA-mediated knockdown ofNRG1in H1793 cells as assessed by quantitative PCR. (f) Knockdown of NRG1 decreased cell proliferation as monitored by IncuCyte confluence analysis. (g) Overexpression of NRG1 induces cell proliferation and migration. Cell proliferation by WST-1 assay (left panel) and cell counting (middle panel) on BEAS-2B cells stably transfected with Lac-Z orCD74-NRG1fusion. Both assays demonstrated that cells expressing theCD74-NRG1fusion had significantly higher proliferation rate at day 3 and 5 (Student’st-testP<0.001 for both time points) as compared with Lac-Z. The right panel represents a cell migration assay after 24 h. BEAS-2B cells expressingCD74-NRG1fusion showed a higher migration rate as compared with Lac-Z (Student’st-testP=0.0014). When TP53 , KRAS and EGFR mutation status or smoking status was included in the multivariate analysis, the number of fusions remained independently associated with poor outcome ( Supplementary Table 6 ). Figure 2: Gene fusion numbers correlates with lung cancer prognosis. Kaplan–Meier analysis for the combined cohort of lung cancer samples ( n =594) with low (0–7) ( n =124), intermediate (8–16) ( n =237), or high (≥17) ( n =233) number of fusions (likelihood ratio test P =0.008). Samples with high number of fusions have worse prognosis (Cox survival analysis P =0.005). Individual Kaplan–Meier analyses with LUAD and LUSC samples are found in Supplementary Fig. 4a,b , respectively. Full size image Private or low recurrence fusions in lung cancer To filter the fusion data and prioritize fusion candidates, we developed a random forest fusion classifier (see Methods). This classifier uses structural and functional annotation features of each fusion to prioritize gene fusion candidates involving exonic regions. Remarkably, our classifier had a true positive recovery rate >90% in two independent validation data sets and automatically recapitulated the intuitive knowledge about the important structural properties defining bona fide fusions ( Supplementary Data 2,3 ). In our fusion data set, the top five features contributing to the fusion classifier were, in decreasing order of importance: fusion type (interchromosomal, intrachromosomal and tandem duplication), sum of the median alignment quality of reads supporting the fusions, number of spanning and encompassing reads across the fusion junction and the cohort-normalized expression value for the 3′-partner gene ( Supplementary Fig. 5 ). Using this classifier, 422 fusions were shortlisted from the entire cohort ( Supplementary Data 4 ). Sixty-four out of 422 fusions (15%) involved kinases (either as 3′- or 5′-partner) including the known ROS1 , RET and ALK fusions: 52 fusions involved oncogenes and 63 involved tumour suppressors ( Supplementary Data 4 ). Moreover, of the fusions involving ‘informative genes’, we found 61 productive in-frame fusions, 63 out-of-frame fusions and 6 promoter fusions. In the KRAS mutant population, a large NSCLC molecular subtype where chemotherapy is the only approved treatment, we identified additional private fusions ( Supplementary Data 4 ). For example, sample pt_lung_A25 contains a driver KRAS G12C and TP53 P72R mutations in addition to fusions with abundant read support. Although the TRAF-interacting protein–inositol hexakisphosphate kinase ( TRAIP-IP6K1 ) fusion results in loss of function of both partners, the SLC12A7-TERT fusion produces an in-frame open reading frame (ORF), where the telomerase domain of TERT is retained and could serve as a potential combinatorial drug target. In another sample, pt_lung_A63, which harboured KRAS G12D , TP53 P72R and ATM E2423K mutations, has a TSC1-SMARCA4 fusion as well. Further pt_lung_C028 with TP53 R248L and SMARCA4 E1056stop mutations also harboured a WASF2 - FGR fusion where the kinase domain of fibroblast growth factor is retained. These three cases are representative examples of private fusions and the additional events that coexist in NSCLC tumours. As our cohort was large enough, we estimated the recurrence of different gene fusions that we classified as molecular, functional or family recurrence. Molecular recurrence were defined as the same 5′- and 3′-partners observed in different samples such as SLC34A2-ROS1 ; functional recurrence refers to when either 5′- or 3′-partner is the same ( CCDC6-RET and KIF5B-RET ); and gene family recurrence correspond to gene fusions in which 5′- or 3′-partners belongs to the same gene family such as FGFR ( FGFR3-TACC3 , FGFR2-CCDC6 and BAG4-FGFR1 ). Functionally recurrent kinase fusions ROS1 , RET and ALK were found in 0.86%, 0.29% and 0.14% across the combined cohort ( Supplementary Data 5 ). Interestingly, in tumours with known driver fusions, the number of ‘classified’ fusions is lower than those without driver fusions (Student’s t -test, t =2.7588, df=5.023, P =0.01985), suggesting their functional importance. Similarly, BCAS3-MAP3K3 , MRC2-MAP3K3 is another example of family recurrence. We observed ‘pathway fusion recurrence’ in which multiple genes in the same signalling pathway are involved in fusions. Interestingly, 10 out of 33 members of the Hippo [28] pathway were identified as fusion partners ( Supplementary Data 6 ). Perturbation of the Hippo pathway in lung cancer The Hippo signalling pathway is highly conserved across species and plays a major role in cell polarity, cell–cell adhesion and contact inhibition [29] . The mammalian homologues of the Drosophila Hippo and Warts core serine–threonine kinases are STE20-like protein kinase ( MST1/2 ) and large tumour suppressor homologue kinase ( LATS1/2 ), respectively. The core kinases regulate the activity and stability of the transcriptional co-activators yes-associated protein 1 ( YAP1 ) and WW domain-containing transcription regulator 1 ( WWTR1 ) through phosphorylation. Unphosphorylated YAP/WWTR1 binds to TEA domain family ( TEAD ) transcription factors in the nucleus to regulate gene expression ( Fig. 3a ). Accessory members of the Hippo pathway such as KIBRA ( WWC1 ), scribbled planar cell polarity ( SCRIB ) and Neurofibromin 2 ( NF2 ) have been shown to activate the core kinases. An increasing number of studies have investigated the Hippo pathway in lung, colorectal, ovarian and liver cancers [29] . Although animal model experiments support a role for the Hippo pathway in tumorigenesis, no evidence for non-synonymous mutations in this pathway has been found in lung cancer. Few somatic or germline mutations discovered in the Hippo pathway genes are found in common human cancers, with NF2 being the only gene known to be inactivated by mutation [29] . We observed novel recurrent NF2 fusions, where retention of only the first exon of NF2 , in both NF2-OSBP2 and NF2-MORC2 fusions result in loss of function of this tumour suppressor gene ( Fig. 3b ) and several fusions involving core members of the Hippo pathway such as LATS1 , YAP1 and WWTR1 (previously known as TAZ ) ( Fig. 3b,c ). We also identified fusions in associate members of the Hippo pathway, including HIPK2 , TAOK1 , TAOK3 , FAT1 , DCHS2 and PTPN14 ( Fig. 3b,c ). Detailed inspection of the fusions revealed two intriguing aspects of these aberrations. Gene fusions in the Hippo pathway tumour suppressor members such as LATS1 , DCHS2 , FAT1 , TAOK1 , TAOK3 , PTPN14 and NF2 ( Fig. 3b,c ) likely abrogated their function by generating truncated proteins. However, fusions involving oncogenic proteins in the Hippo pathway such as WWTR1 , YAP1 and HIPK2 potentially retained their crucial functional domains Fig. 3c ). Furthermore, we investigated the presence of additional genetic aberration in the index fusion samples and noticed that the vast majority lack known driver mutations (10 out of 14) ( Supplementary Data 6 ). Using cbioportal ( http://www.cbioportal.org ), we discovered copy number loss and associated low mRNA expression of FAT1 in the index fusion sample ( Supplementary Fig. 6a ) and copy gain and elevated expression of YAP1 in the sample harbouring YAP1 fusion ( Supplementary Fig. 6b ). These observations suggest that gene fusions are a novel mechanism of altering the Hippo pathway genes potentially promoting a transforming phenotype. Taken together, the fusion landscape in lung cancer is highly heterogeneous and characterized by low recurrence and private fusions ( Supplementary Data 5 ). Despite this heterogeneity, gene fusions could still be functionally relevant in lung cancers by affecting several members of common pathways such as those of the Hippo signalling cascade we observed here. Figure 3: Gene fusions among the Hippo pathway genes in lung cancer. ( a ) Schematic representation of core and associate members of the Hippo pathway adapted from Harvey et al . [29] Potential tumour suppressors are represented in green, whereas potential oncogenes are indicated in red. Phosphorylation of YAP or TAZ by LATS retains them in the cytoplasm and hinders their transcriptional regulation. ( b ) Fusions in putative oncogenes of the Hippo pathway. ( c ) Fusions in putative tumour suppressors of the Hippo pathway. For all fusion schematics represented, the wild-type Hippo pathway protein domain structure is presented first, numbers indicate total amino acids and domain names are abbreviated. Red arrows show the fusion junctions and red # symbol indicate protein truncation due to out-of-frame ORFs from fusion transcript analysis. The schematic of the previously reported TAZ -CAMTA1 fusion in epithelioid hemangioendothelioma (EH) [42] is also displayed. Protein abbreviations: MST1/2, STE20-like protein kinase; LATS1/2, large tumour suppressor homologue kinase; YAP1, Yes-associated protein 1; WWTR1, ww-domain containing transcription regulator 1; TEAD, TEA-domain family; HIPK2, homeodomain interacting protein kinase 2; TAOK1/3, TAO kinase; FAT1, FAT atypical cadherin 1; DCHS2, dachsous cadherin-related 2; PTPN14, protein tyrosine phosphatase, non-receptor type 14. Domain abbreviations: B4, Band 4.1 homologues; FERM_C, FERM C-terminal PH-like domain; S_TKc, serine/threonine protein kinases, catalytic domain; PTPc, protein tyrosine phosphatase, catalytic domain; CA, cadherin repeats; FIB, fibrinogen; FBG, fibrinogen-related domains; WW, domain with 2 conserved Trp (W) residues; TID, TEAD interacting domain; TAD, transactivation domain; ANK,ankyrin repeats; IQ, short calmodulin-binding motif; EGF, epidermal growth factor-like domain; ZnFC2H2, zinc finger; TM, transmembrane domain. Full size image Inactivating fusions of NF1 in lung cancer Next, our integrative analysis combining fusion and mutation status revealed a total of 33 samples with aberrations in NF1 gene such as truncating fusions— GOSR1-NF1 , NLK-NF1 and NF1-PSMD11 —or deleterious mutations—non-sense, frame shift or splice site ( Fig. 1 , Fig. 4a and Supplementary Table 7 ). The fusions and mutations were observed in both LUAD and LUSC predominantly in driver-negative samples (27 out of 33). Loss of NF1 promotes cell proliferation by de-repressing the mammalian target of rapamycin pathway in a RAS-, phosphoinositide 3-kinase-dependent manner [30] , [31] . The fusion architecture renders the tumour suppressor NF1 inactive by either truncating ORFs ( GOSR1-NF1 and NLK-NF1 ) or by destroying its functional domains ( NF1-PSMD11 ) ( Fig. 4a,b ), indicating an alternate mechanism for NF1 inactivation in lung cancers besides somatic mutations [4] . To assess additional NF1 destructive fusions in lung cancer, we did a comprehensive analysis assessing fusion junctions involving either exons or introns, and found two additional events of NF1-DRG2_Antisense and NF1-MYO15A_Antisense present in the LS2 sample ( Fig. 4a,b ). The read evidence suggests genomic deletion as the mechanism for the NF1 fusions, except in sample LS2 where centromeric inversion may be the underlying aberration ( Fig. 4b ). Importantly, 20 out 29 mutated NF1 samples and all NF1 truncating fusions were observed in samples without known drivers, accounting for 6.2% (24/386) of this subpopulation. Interestingly, two samples had fusions accompanying somatic mutations in NF1 , potentially altering both the alleles of this tumour suppressor gene ( Supplementary Table 7 ). Figure 4: Inactivating gene fusions of NF1 in lung cancer. ( a ) NF1 protein schematic and the observed fusion breaks (red arrows) in the index cases are displayed on top. Recurrent NF1 fusions with partners ( GOSR1 , PSMD11 , NLK , DRG2 antisense and MYO15A antisense) resulted in loss of the NF1 gene as illustrated by the corresponding fusion protein structure below. Index samples are indicated in parenthesis and the numbers over the protein schematic indicate total amino acids. Red # symbol indicate protein truncation due to out-of-frame ORFs from fusion transcript analysis. ( b ) UCSC browser view of genomic location of NF1 gene and its fusion partners (top). Schematic representation of various NF1 rearrangements on chromosome 17 identified in lung cancer (bottom). Full size image Exon skipping and coincident splice site mutations in c-MET Recently, a significant per cent of driver-unknown lung cancer samples have been shown to harbour fusions involving ALK , ROS1 and RET [19] , [23] kinases, and an activating exon skipping in the c-MET oncogene [23] . Our analysis revealed 1.3%, 0.52% and 0.26% fusions involving ROS1 , RET and ALK , respectively, among LUAD and LUSC with unknown driver. We detected c-MET exon-14 skipping in 15 samples, 14 of which occurred in driver-unknown samples, a 3.6% (14/386) recurrence rate in this subpopulation ( Fig. 5 ). Importantly, in 5 out of 15 samples, the skipping of c-MET exon-14 is probably caused by a mutation affecting the splice donor site adjacent to the amino acid position D1010 as previously described [32] . Our RNASeq data also validated the reported c-MET exon-skipping event in the H596 cell line [23] . Figure 5: Recurrent activating MET exon-skipping events. Right panel: an activating MET exon-14 skipping event was observed in a total of 15 tissue samples across all three cohorts. The total reads supporting each splice variant exon13–14 (blue), exon13–15(red) and exon14–15 (green) are represented in the bar plot on the right. In 5 out of 11 TCGA samples where DNA mutation data were available, skipping of MET exon-14 was accompanied by a mutation affecting the splice donor site adjacent to position D1010 (illustrated inset on the right). In addition, one sample harboured a non-sense mutation g.chr7:116412024C>Gp.Y1003*, which accompanied exon-14 skipping. Left panel: IGV browser view of splice site deletions/mutations in the corresponding samples. Full size image Outlier kinase expression in lung cancer Next, integrative analysis combining the mutation, fusion and gene expression data revealed outlier expression information in the context of fusions and mutations per sample. Focusing on kinase genes for example ROS1 , we noticed six samples across the combined cohort with outlier ROS1 expression that lacked any evidence for ROS1 fusions. A similar phenomenon was also observed in cases with FGFR3 outlier expression. Intriguingly, tumours showing outlier expression of ROS1 and FGFR3 are almost exclusively driver unknown samples without evidence of fusions (Fisher’s exact test, P =0.004 and P =0.086, respectively, Fig. 1 ). Fluorescence in-situ hybridization analysis of ROS1 ( n =1) and RET ( n =3) outlier index cases did not detect any gene rearrangements. Hence, although the mechanism of overexpression remains to be determined, the outlier kinase expression may act as oncogenic drivers and be potentially actionable. Recurrent NRG1 rearrangements with novel fusion partners in lung cancer Remarkably, we noted functionally recurrent gene fusion where the common 3′-gene neuregulin 1 ( NRG1 ) was fused to various 5′-partners ( Fig. 6a and Supplementary Table 8 ) CD74-NRG1 , RBPMS-NRG1 , WRN-NRG1 and SDC4-NRG1 , in both LUAD and LUSC samples. Importantly, CD74-NRG1 fusion variant was recently identified by three independent groups [20] , [21] , [22] . Although CD74-NRG1 , SDC4-NRG1 and RBPMS-NRG1 fusion events resulted in the production of chimeric proteins, the WRN-NRG1 fusion results in the overexpression of full-length NRG1 regulated by the WRN gene promoter. As a member of EGF ligand family, NRG1 transduces its signal through the HER/ErbB family receptor tyrosine kinases [33] , [34] . NRG1 functional domains include kringle-like, immunoglobulin-like domain and the EGF domain located in the carboxy-terminal region [33] . Notably, the EGF domain is essential for receptor interaction [35] and is preserved in all the NRG1 fusions identified ( Fig. 6a ). All NRG1 fusion index lung samples were found in samples without known-driver mutations and displayed NRG1 outlier expression in the tumour but not matching normal tissue ( Figs 6b,c ). Strikingly similar to the pattern described above for the known receptor kinases fusions, we noticed NRG1 outlier expression in both index fusion samples ( n =4) and an independent set of known driver aberration negative cases ( n =10; Supplementary Table 8 ). Among the lung cancer cell line RNASeq data, H1793 exhibited the highest NRG1 transcript expression ( Fig. 6d and Supplementary Fig. 2 ). At 70% knockdown with two independent NRG1 small interfering RNAs ( Fig. 6e ), H1793 cell proliferation rate was affected as assessed using cell growth assays ( Fig. 6f ). Conversely, on stable overexpression of the CD74-NRG1 fusion protein in normal lung BEAS-2B cells, we observed significant increase in cell proliferation, migration ( Fig. 6g and Supplementary Fig. 7a ) and an altered morphology relative to LacZ controls ( Supplementary Fig. 7b,c ). CD74-NRG1 overexpression induces epithelial to mesenchymal transition (EMT) as evidenced by increased VIM and SNAIL protein expression and decreased CDH1 level by western blot analysis ( Supplementary Figs 7d and 9 ). We next performed gene expression profiling of CD74-NRG1 and LacZ control cells, to identify affected biological pathways. Significant analysis of microarrays showed overexpression of several EMT markers such as VIM , ZEB1 , ZEB2 , FZD7 , TWIST1 , VCAN and CHD2 , and underexpression of RGS2 and CDH1 among others, further supporting the EMT phenotype in CD74-NRG1 -positive cells ( Supplementary Data 7 ). Vimentin, ZEB1 and ZEB2 were overexpressed more than four fold, while CDH1 and RGS2 were among the most underexpressed genes ( Supplementary Figs 7e and 8a ). Gene set enrichment analysis identified downregulation of cell adhesion ( Supplementary Fig. 8b ) and upregulation of the SRC and ERBB pathways ( Supplementary Fig. 8c and d ) in CD74-NRG1 cells. We examined both total and phosphorylated ERBB3, a receptor known to bind NRG1, and observed a substantial decrease in total ERBB3 on overexpression of CD74-NRG1, which was also reflected in its phosphorylated form as compared with LacZ control ( Supplementary Figs 8e and 9 ). Despite the observed decrease in total ERBB3 in the fusion-expressing cells, phospho-ERBB3 was still detectable ( Supplementary Figs 8e and 9 ). Total ERBB3 decrease on exposure to NRG1 has been previously demonstrated in MCF-7 (ref. 36 ) and also in H568 lung cells on CD74-NRG1 overexpression [20] . In addition, we observed increased levels of phosphoERK (1.95-fold) and phosphoJNK1 (5.5-fold) relative to LacZ control ( Supplementary Figs 8e and 9 ), potentially promoting the oncogenic phenotype in NRG1 fusion-overexpressing cells. Finally, we examined other cancer types for NRG1 fusions and discovered one additional RAB2IL1-NRG1 fusion in the TCGA ovarian cancer RNASeq data. As observed in lung cancer, the functional EGF domain is retained in RAB2IL1-NRG1 and the fusion index case exhibited outlier NRG1 expression ( Fig. 6a,b ). Altogether, NRG1 is perturbed ( NRG1 fusions and/or outlier expression) in 3.9% (15/386) of driver-unknown samples, supporting a causal role for NRG1 in this lung cancer patient subpopulation. Figure 6: Recurrent NRG1 rearrangements in lung cancer. ( a ) Recurrent fusions involving NRG1 as a 3′-partner were detected in lung adenocarcinoma and lung squamous carcinoma in the three cohorts included in this study. Schematic representation of functional domains present in the NRG1 fusion proteins namely CD74-NRG1 ; RBPMS-NRG1 (LUAD), WRN-NRG1 (LUSC), SDC4-NRG1 (LUSC) and RAB2IL1-NRG1 (ovarian cancer from TCGA) compared with the wild-type NRG1 (top). The receptor-binding EGF domain is preserved in all fusions. TM, transmembrane domain; RRM domain; IGc2 domain; SEC2P domain. ( b ) Analysis of RNASeq expression values revealed outlier NRG1 mRNA expression in all index cases (large blue dots) within each cohort. ( c ) High NRG1 mRNA expression driven by the fusion event in the index tumour tissue compared with matched normal, in both an LUAD patient in the University of Michigan and Seoul cohorts. ( d ) Box plot showing outlier expression of NRG1 in H1793 in the University of Michigan lung cell line cohort. ( e ) Two independent small interfering RNA-mediated knockdown of NRG1 in H1793 cells as assessed by quantitative PCR. ( f ) Knockdown of NRG1 decreased cell proliferation as monitored by IncuCyte confluence analysis. ( g ) Overexpression of NRG1 induces cell proliferation and migration. Cell proliferation by WST-1 assay (left panel) and cell counting (middle panel) on BEAS-2B cells stably transfected with Lac-Z or CD74-NRG1 fusion. Both assays demonstrated that cells expressing the CD74-NRG1 fusion had significantly higher proliferation rate at day 3 and 5 (Student’s t -test P <0.001 for both time points) as compared with Lac-Z. The right panel represents a cell migration assay after 24 h. BEAS-2B cells expressing CD74-NRG1 fusion showed a higher migration rate as compared with Lac-Z (Student’s t -test P =0.0014). Full size image Increased understanding of lung cancer has resulted in the identification of therapeutic molecular targets and development of relevant targeted therapies. For example, EGFR -activating mutations in exons 18, 19 and 21 are now routinely assessed in tumour biopsies before treatment with gefitinib or erlotinib; the response rate is nearly 70% in mutation-positive advanced NSCLC [37] . Further, fusions involving ROS1 , ALK and RET [15] , [16] , [38] tyrosine kinases are identified primarily in younger patients with LUAD and without known driver mutations or significant smoking history. Despite the low fusion frequency, clinical trials for ALK-positive lung cancer patients have shown higher response rate and longer progression-free survival when treated with crizotinib, a drug targeting ALK, relative to chemotherapy [39] , [40] . These results support targeting specific molecular aberrations in patients’ tumours. In this study, RNA sequencing was used to characterize the fusion landscape of NSCLC in an unbiased manner. We find the fusion landscape highly heterogeneous dominated by private and low recurrence fusions, with a greater number of fusions per sample detected in LUSC than LUAD on average (Student’s t -test, P <2.2e−16). No statistically significant difference, with respect to any other clinical characteristics such as smoking history or disease stage, was observed ( Supplementary Tables 3–5 ). Importantly, a higher number of fusions were independently associated with poor overall survival ( Fig. 2 and Supplementary Table 5 ), after adjusting for histological subtype, age, gender, disease stage and TP53 , KRAS and EGFR mutation status ( Supplementary Table 6 ). As RNA sequencing becomes widely adopted for profiling transcript expression and gene fusion detection, our results suggest that the number of fusions could also be used as an independent prognostic marker in lung cancers. Our analysis of functionally recurrent fusions identified aberrations in multiple members of the Hippo pathway. This evolutionarily conserved pathway regulates tissue growth and cell fate, and has been thought to play an important role in cancer [28] . Functional studies conducted in mouse models showed that knockdown of tumour suppressor or overexpression of oncogene members of the pathway-induced tumour formation [29] . Furthermore, two recent reports identified recurrent fusions involving WWTR1 , an oncogene member of the Hippo pathway and CAMTA1 in epithelioid hemangioendothelioma [41] , [42] . The previously reported WWTR1 fusion and the one in our study ( WWTR1-SLC9A9 ) ( Fig. 3 ) have identical WWTR1 gene breakpoints, whereby the functional WW domain of WWTR1 is retained in both fusion events. We also observed fusions involving 3 out of 13 core members and 7 out of 20 associate members of the Hippo pathway ( Fig. 3 ). A recent study has demonstrated the role of STK11 (also called LKB1) in regulating the core Hippo kinases through Scribble [43] . The tumour suppressor STK11 is frequently inactivated in lung cancer ( Fig. 1 ), which is associated with YAP activation. This discovery now vastly expands the incidence of the Hippo pathway aberration in lung cancers. Interestingly, gene fusions in the Hippo pathway tumour suppressor members appear to abrogate their function by generating truncated proteins, while fusions involving oncogenic proteins in the Hippo pathway retain their crucial functional domains ( Fig. 3 ). Taken together, our data now present novel evidence for the involvement of the Hippo pathway in lung cancer. The recurrent tyrosine kinase fusions mentioned earlier were found almost exclusively in LUAD not harbouring known fusions and have not been previously identified in the LUSC subtype. Here we observed a recurrent fusion with NRG1 as 3′-partner ( CD74-NRG1 , RBPMS-NRG1 and WRN-NRG1 ) in both LUAD and LUSC ( Fig. 6 ). NRG1, a growth factor that interacts with the HER/ErbB receptor tyrosine kinases, is expressed in a subset of cancers, including breast, lung and other cancers [44] . CD74 is a known 5′-fusion partner of ROS1 kinase in lung cancer. Although CD74-NRG1 and WRN-NRG1 fusions contain the signal peptide and type II transmembrane domain required for NRG1 localization to the plasma membrane, cellular location of RAB2IL1-NRG1 and RBPMS-NRG1 fusion proteins is uncertain. However, of the 20 NRG transcript variants (transcribed from NRG 1–4) reported, several lack the N-terminal signal sequence required for membrane localization and transport to the extracellular space. In these instances, an internal hydrophobic amino acid stretch is speculated to substitute for the N-terminal signal sequence [33] , [35] . In addition, we identified a novel SDC4-NRG1 fusion in two samples added to the TCGA cohort after our data freeze. The SDC4-NRG1 fusion produces a secretory NRG1 protein due to the signal peptide contributed by SDC4 protein. This observation suggests that incidence of NRG1 aberrations in lung cancer is likely to increase as more samples are characterized. Remarkably, NRG1 fusions are present in tumours without known-driver events ( Fig. 1 and Supplementary Table 8 ) and the index samples display outlier NRG1 expression ( Fig. 6 ), similar to oncogenic fusions such as ROS1 . Moreover, we found additional cases of NRG1 outlier expression in samples without known driver mutations, suggesting a potential role for NRG1 in those samples. We demonstrated that abrogating NRG1 expression affects cell proliferation ( Fig. 6 ) and, more importantly, we showed that human bronchial cells stably expressing CD74-NRG1 promoted proliferation and migration ( Fig. 6 ). Three independent studies have very recently associated CD74-NRG1 fusions with mucinous LUAD subtype [20] , [21] , [22] . We further examined our samples and discovered that HNF4A , a recently characterized biomarker for mucinous LUAD [45] , showed highest expression in our CD74-NRG1 index case, providing independent support for association of NRG1 gene fusions with mucinous LUAD. Interestingly, the SDC4-NRG1 index sample with the highest NRG1 outlier expression ( Fig. 6b , NRG1 expression: 380 fragments per-kilo base per million, higher than the cell line H1793) did not show high HNF4A expression, suggesting that NRG1 fusions with partners other than CD74 are perhaps more prevalent in non-mucinous LUAD . NRG1 rearrangements have also been detected using FISH in breast cancer cell lines [46] . Moreover, NRG1 overexpression was recently demonstrated in a subset of breast clinical tumour samples and was mutually exclusive with HER2 mutations [47] . These observations together with our results from lung and ovarian cancers suggest that NRG1 rearrangements are recurrent and probable drivers of various cancers types. The therapeutic targeting of NRG1-ERBB autocrine loop was previously suggested [48] , and recently blocking NRG1 and other ligand-mediated HER4 signalling was shown to enhance the magnitude and duration of the chemotherapeutic response of NSCLC [49] . Therefore, the characterization of all NRG1 fusions presented in this study, as well as the common signalling pathways activated in both fusion and outlier expression index samples, could further elucidate NRG1 mechanism of action and reveal further therapeutic opportunities. Our integrative analysis combining mutation and fusion status extended previous observations of c-MET exon skipping and NF1 truncating mutations. We detect novel truncating fusions involving several tumour suppressor genes such as NF1 , NF2 , TP53 (data not shown), LATS1 , DCHS2 , FAT1 , SMARCA4 , TAOK1 and TAOK3 among others. These results highlight gene fusions as potentially common and a previously underappreciated mechanism for loss of function of many tumour suppressor genes. In summary, the Hippo pathway fusions (2.6%), NRG1 fusion/outlier expression (3.9%), NF1 truncating mutations/fusions (6.2%) and c- MET exon skipping (3.6%) account for ~16% of driver-unknown lung cancer cases and expanding the repertoire of lung cancer molecular subtypes. The previously documented success of targeted therapies against low-recurrence oncogenic fusions and the heterogeneity of the fusion landscape, demonstrated in this study, reinforce the demand for personalized molecularly targeted drug therapies in lung cancer. Sample acquisition and total RNA isolation We collected tumour samples from 67 LUAD, 36 LUSC and 9 LCLC patients, along with 6 matched normal lung tissue samples following surgery at the University of Michigan. The recruitment of subjects and informed consent were reviewed and approved by our Institutional Review Board. The publically available data set from TCGA was downloaded using the TCGA portal and the Seoul data from dbGAP. Formalin-fixed, paraffin-embedded (FFPE) sections from 11 adenoid cystic carcinoma samples were from IRCCS AOU San Martino-IST, Genoa, Italy. The 24 lung cell lines were purchased from American Type Culture Collection and cultured following their media and growth conditions. Total RNA from frozen tissues or cell lines were isolated using miRNeasy mini kit (Qiagen, Valencia, CA), while RNA was isolated from FFPE sections using FFPE RNAeasy kit (Qiagen). Only high-quality RNA from frozen sections and cell lines with RNA integrity number >8.0, on 2100 Bioanalyzer analysis (Agilent, Santa Clara, CA) were subjected to RNA sequencing ( Supplementary Methods ). Preparation of RNASeq libraries and sequencing Transcriptome libraries were prepared following a previously described protocol for generating strand-specific RNASeq libraries with slight modifications [50] ( Supplementary Methods ). Libraries were next size selected in the range of 350 bp after resolving in a 3% Nusieve 3:1 (Lonza, Basel, Switzerland) agarose gel and DNA recovered using QIAEX II gel extraction reagent (Qiagen). Libraries were barcoded during the 14-cycle PCR amplification with Phusion DNA polymerase (New England Biolabs, Ipswich, MA) and purified using AMPure XP beads (Beckman Coulter, Brea, CA). Library quality was estimated with Agilent 2100 Bioanalyzer for size and concentration. The paired-end libraries were sequenced with Illumina HiSeq 2000 (2 × 100bases, read length). Reads that passed the filters on Illumina BaseCall software were used for further analysis. The data have been deposited to Sequence Read Archive (SRA) under the SRA accession number SRP048484. Cloning of CD74-NRG1 fusion and functional assays CD74-NRG1 fusion transcript was amplified from the index lung cancer sample tissue complementary DNA with forward 5′- CACCATGCACAGGAGGAGAAGCAGGAGCTGT -3′ and reverse primers 5′- TTCAGGCAGAGACAGAAAGGGAGTGGA -3′ using Hi-fidelity polymerase (Qiagen). The PCR product was gel purified and cloned into pLenti-TOPO cloning vector (Invitrogen, Carlsbad, CA) and Sanger sequencing verified. The control LacZ or C-terminal V5-tagged CD74-NRG1 constructs were transfected into the normal lung epithelial BEAS-2B cells. The stable cells were generated following selection in BEBM media (Lonza) containing 3 μg of blasticidin (Invitrogen). For proliferation assays, 50,000 cells were plated in 12-well plates and grown in regular media. Cells were harvested by trypsinization and counted manually at indicated time points. All assays were performed in quadruplicates. For migration assays, stable cells were re-suspended in medium without growth factors, then seeded at 50,000 cells per well into Boyden chambers (8 μm pore size, BD Biosciences) and were incubated for 24 h in a humidified incubator at 37 °C, 5% CO 2 atmosphere. The bottom chamber contained medium with growth factors as chemo-attractant. The top non-migrating cells were removed with a cotton swab moistened with medium and the lower surface of the membrane was stained with Diff-Quick Stain Set (Siemens). The number of cells migrating to the basal side of the membrane was visualized with an Olympus microscope at × 20 magnification. Pictures of five random fields from four wells were obtained and the number of stained cells was quantified. Sequence alignment and analyses Sequence alignment was performed using the Tuxedo pipeline: Bowtie2 (Bowtie2/2.0.2) and Tophat2 (TopHat/2.0.6) [51] . Fusion calling was performed with TopHat-fusion (THF) [51] on the UMICH, TCGA and Seoul cohorts. Additional details and parameter values used for sequence alignment and fusion calling are provided in the Supplementary Methods . Fusion annotation and lung cancer fusions database A database of fusions in lung cancers was developed, and for each fusion structural and functional annotations were recorded. The structural information corresponds to characteristics such as fusion type (interchromosomal, intrachromosomal, tandem duplication), number of spanning and encompassing reads and median alignment quality of reads that support 3′- and 5′-gene, among others (see Supplementary Methods ). The functional annotation corresponds to features such as kinase status, oncogene status and tumour suppressor status among others. Moreover, the gene expression of the 5′- and 3′-partner genes was calculated in fragments per-kilo base per million using Cufflinks [52] and stored in the database. Furthermore, the outlier sum score [53] was independently calculated for the expression of both 5′- and 3′-partners, to identify fusion cases for which the 3′-gene partner was highly expressed relative to its median expression in the cohort. Overexpression of the 3′-partner as a consequence of gene fusions has been observed in well-known fusions such as TMPRSS2-ERG and others [54] . Finally, we also recorded the mutation status for each patient, allowing us to classify each patient as ‘driver positive’ or ‘driver negative’ according to mutation status of well-known cancer-related genes ( Supplementary Methods ). Fusions classifier All fusion-calling algorithms produce a significant number of false-positive fusions when applied on RNASeq data. Many of these spurious fusions are due to diverse and difficult-to-model bioinformatics, sequencing and biological factors such as template switching, and chimeric events associated with amplicon regions among others [55] , [56] , [57] . Therefore, we developed a classifier to prioritize fusions for follow-up based on the structural and functional features collected for each fusion, which were described above and stored in our fusion’s database. THF called 31,304 fusions across the combined cohort, making the task of separating false-positive fusions from potentially true ones far from trivial. We first reasoned that functional fusion proteins have ORFs; therefore, fusions in which the exon of one gene is fused to the intron of another, or two introns are fused together, would not produce fusion products with ORFs. This first-level filtering reduced to 6,465 the number of fusions to classify. Next, we reasoned that fusions found in normal samples, fusions involving pseudogenes, lincRNAs, or antisense transcripts and fusions for which the median alignment quality of reads supporting any of the gene partners was equal to zero (indicating multi-mapping) are potentially false positives, and these were excluded from downstream analysis. This second-level filtering reduced to 4,990 the number of fusions called by THF. As assessing the quality of each one of those fusions manually is impractical, we built a random forest classifier to prioritize what fusions to follow up out of those 4,990 gene fusions. For the classification step, we trained a random forest classifier with 10,000 trees using the structural, functional and expression features described above ( Supplementary Methods ). True-positives examples were selected from the TCGA, Seoul and UMICH cohorts. On one hand, the examples chosen from the TCGA and Seoul cohorts correspond to well-known fusions involving ALK, RET and ROS1 kinases. On the other, the examples chosen from the UMICH cohort correspond to fusions called by at least two independent algorithms, carefully curated manually and validated by PCR ( Supplementary Data 4 ). False-positive examples were identified representing different types of spurious fusions: for example, overlapping genes, and fusions involving highly expressed genes such as ribosomal proteins among others. After applying the classifier, we obtained 422 high-quality gene fusions. Taken together, our approach allowed us to efficiently prioritize the initial set of 31,304 fusions reported by THF, filtering out potential false positives. Finally, ORF prediction and protein domain retention analysis were performed in recurrent fusions or biologically interesting fusions found in this final set of 422 fusions. An additional advantage of using a classifier to determine the potential true fusions, as opposed to hard filters defined a priori , is that we can learn those features or rules from the data itself. In our data set, the top five features that contributed the most for the random forest classifier were, in decreasing order of importance, fusion type (interchromosomal, intrachromosomal, tandem duplication), sum of the median alignment quality of both gene partners, number of reads spanning and encompassing reads across the fusion junction and the cohort normalized expression value of the 3′-gene ( Supplementary Fig. 5 ). Two additional sets of true fusions were left out of the training data set to calculate the recovery rate. First, a set of 11 fusions called in the Seoul cohort [19] and validated by PCR by the same authors, and a second set of 15 fusions called in the UMICH cohort by THF and validated by PCR. In the first of these data sets, our classifier recovered 10 out of 11 true fusions for a 90.1% recovery rate ( Supplementary Data 2 ). In the second set, the classifier recovered 14 out of 15 validated fusions for a 93.3% recovery rate ( Supplementary Data 3 ). How to cite this article : Dhanasekaran, S. M. et al . Transcriptome meta-analysis of lung cancer reveals recurrent aberrations in NRG1 and Hippo pathway genes. Nat. Commun. 5:5893 doi: 10.1038/ncomms6893 (2014).